Genome sequences of wild and domestic bactrian camels Bactrian camels serve as an important means of transportation in the cold desert regions of China and Mongolia. Here we present a 2.01 Gb draft genome sequence from both a wild and a domestic bactrian camel. We estimate the camel genome to be 2.38 Gb, containing 20,821 protein-coding genes. Our phylogenomics analysis reveals that camels shared common ancestors with other even-toed ungulates about 55–60 million years ago. Rapidly evolving genes in the camel lineage are significantly enriched in metabolic pathways, and these changes may underlie the insulin resistance typically observed in these animals. We estimate the genome-wide heterozygosity rates in both wild and domestic camels to be 1.0 × 10 −3 . However, genomic regions with significantly lower heterozygosity are found in the domestic camel, and olfactory receptors are enriched in these regions. Our comparative genomics analyses may also shed light on the genetic basis of the camel's remarkable salt tolerance and unusual immune system. Wild bactrian camels ( Camelus bactrianus ferus ) are the lone survivors of the old world camels [1] . At present, their total number is only 730–880, less than that of the giant pandas [2] . They live in northwestern China and southwestern Mongolia, especially the Outer Altai Gobi Desert. Considered critically endangered by the International Union for Conservation of Nature, wild bactrian camels are protected under both the Convention on International Trade in Endangered Species of Wild Fauna and Flora and domestic legislations in China and Mongolia. The archaeozoological record shows that fully domesticated bactrian camels were present in the third millennium BC and subsequently spread into much of Central Asia [3] . However, our knowledge about the origins and migration history of domestic camels remains inconclusive. To adapt to the harsh conditions—cold, hot, arid, and poor grazing—of deserts or semi-deserts, camels have acquired many special abilities and attributes. They can store energy in their humps and abdomen in the form of fat, enabling them to survive long periods without any food or water [4] . The camel’s body temperature may vary from 34 to 41 °C throughout the day [5] . Blood glucose levels in camels are twice those of other ruminants [6] . Camels tolerate a high dietary intake of salt, consuming eight times more than cattles and sheep [7] , yet they do not develop diabetes or hypertension. The Camelidae family are the only mammals that can produce heavy-chain antibodies (HCAbs), a special form of immunoglobulin that lacks the light chain, in contrast to conventional antibodies (Abs) [8] . HCAbs are smaller and more stable, offering particular advantages in various medical and biotechnological applications. In this study, we sequenced the genomes of both wild and domestic bactrian camel, to better understand the history of their evolution and domestication, and to provide a resource for research into the genetic mechanisms that enable camels to survive extreme environments. Genome sequence We sequenced the genomes of an 8-year-old wild male bactrian camel named ‘Naran’ from the wild bactrian camel nature reserve of Altai province, Mongolia (‘wild camel’ hereafter, Supplementary Fig. S1 ) and a 6-year-old male Alashan bactrian camel from Inner Mongolia, China (‘domestic camel’ hereafter, Supplementary Fig. S2 ). For the wild camel genome, four paired-end/mate-pair sequencing libraries were constructed with insert sizes of 500 bp, 3 kb, 10 kb and 20 kb. For the domestic camel genome, only libraries with shorter insert size of 500 bp were constructed ( Supplementary Table S2 ). We assembled the short reads obtained from the wild camel genome sequencing using SOAPdenovo [9] . The reads with the insert size of 500 bp were first assembled into contigs. Then the contigs were joined into scaffolds with reads from the shortest to the longest insert size. In total, we obtained 120,352 scaffolds, including 13,544 scaffolds longer than 1 kb and 3,453 longer than 10 kb. 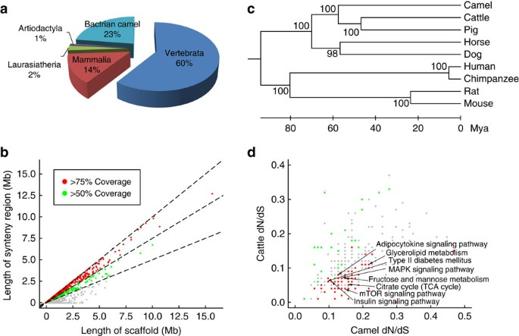Figure 1: Genomic comparison between bactrian camel and other animals. (a) Proportion of shared orthologs between bactrian camel and animals inVertebrata(chicken and zebrafish; NCBI genome accession codes GCF_000002315.3 and GCF_000002035.4),Mammalia(human, chimpanzee, mouse and rat; NCBI genome accession codes GCF_000001405.21, GCF_000001515.5, GCF_000001635.20 and GCF_000001895.4),Laurasiatheria(dog and horse; NCBI genome accession codes GCF_000002285.3 and GCF_000002305.2) andArtiodactyla(cattle and pig; NCBI genome accession codes GCF_000003055.4 and GCF_000003025.5). (b) Length of syntenic regions on each scaffold (Mb, million base pairs). Coverage is calculated as the length of syntenic region divided by the length of scaffold. Scaffolds with coverage >75%, >50% and <50% are represented by red, green and grey dots, respectively. (c) Supertree inference for nine mammals. The topology was evaluated by input tree bootstrap percentages. Distances are shown in millions of years. (d) Points represent pairs of medians of dN/dS ratios in camels and in cattle by KEGG pathways. Pathways in which rapidly evolving genes are significantly enriched (FDR<0.05) in camels and cattle are coloured in red and green, respectively. MAPK, mitogen-activated protein kinase; mTOR, mammalian target of rapamycin; TCA, tricarboxylic acid cycle. The N50 length of the scaffolds longer than 1 kb is 2.00 Mb ( Table 1 ). We remapped the usable reads to the scaffolds and obtained an average effective depth of 76 × and 24 × for the wild and the domestic camel genomes, respectively ( Supplementary Table S3 ). Using the frequency distribution of 17-mer in the reads ( Supplementary Fig. S3 ), we estimated the camel genome size to be 2.38 Gb. This is close to the camel genome size (2.02–2.40 Gb) calculated based on haploid DNA contents ( C values) ( Supplementary Table S4 ). Table 1 Statistics of wild camel genome assembly. Full size table The genome sequences show that 34% of the bactrian camel genome are repetitive DNAs ( Supplementary Table S5 ). This percentage is lower than that in human (>50%) [10] , horse (46%) [11] or cattle (48%) [12] , but close to that in mouse (35%) [13] or dog (34%) [14] . Most of the repetitive DNAs are transposon-derived repeats. Long interspersed elements cover 19% of the whole genome, comparable to human (21%), mouse (19%), horse (20%) and cattle (23%). In contrast, the percentage of short interspersed elements is lower in bactrian camel (4%) than in human (13%), mouse (8%), horse (7%) and cattle (18%). This is likely one of the reasons that the bactrian camel has a smaller genome size than other mammals, for example, human (2.9 Gb) [10] , mouse (2.5 Gb) [13] , horse (2.7 Gb) [11] and cattle (2.9 Gb) [12] . Especially, although copies of ALU repeats appear frequently in primate genomes [15] , none exist in the bactrian camel genome. In addition, 244,141 simple repeats (microsatellite) loci were identified in the camel genome ( Supplementary Table S5 ), which should be useful in quantitative trait locus mapping or marker assistant selection in camels. Gene content and annotation We annotated the camel genome using two ab initio gene finders: Augustus [16] and GenScan [17] . We also utilized the homology-based method, comparing it with several other mammalian genomes, including human, chimpanzee, mouse, rat, dog, horse and cattle, as well as the published expressed sequence tag data [18] of dromedary camels. Combining these two methods, we predicted 20,821 bactrian camel genes, averaging eight exons and 1,322 bps coding region (CDS) per gene. Notably, the GC content of the CDS region is 52%, significantly higher than that of the whole genome (41%). Similar differences were observed in other mammals such as pig (50% versus 40%) [19] . Among the camel genes, 12,050 were annotated to at least one term in Gene Ontology (GO) [20] ( Supplementary Fig. S4 ), and 4,750 genes were annotated to 288 KEGG pathways [21] . According to the InterProScan [22] annotation ( Supplementary Fig. S5 ), the most common protein domains found in the camel genome are immunoglobulin-like domains, consistent with a previous report [18] . The largest protein family identified from the camel genome is the rhodopsin-like G protein-coupled receptor family, which, with 1,011 members, is well-known for controlling the signalling pathways of many biological and physiological processes such as feeding, reproduction and behaviour. Genome evolution HomoloGene [23] was used to examine the conservation of gene repertoires among bactrian camels and other vertebrate species. A total of 16,065 camel genes were grouped into 12,536 orthlogous families, of which 12,521 genes are conserved in vertebrates and 2,912 in mammals ( Fig. 1a ). A total of 4,756 unique genes were found in bactrian camels, among which 3,774 genes do not have GO annotations. Using the identified orthologs as anchor points, we constructed the syntenic maps between the camel and other mammalian genomes ( Supplementary Table S6 ). In total, we identified more than 1,100 syntenic blocks in the camel genome, which cover 12,965 orthologous camel genes ( Fig. 1b ). Figure 1: Genomic comparison between bactrian camel and other animals. ( a ) Proportion of shared orthologs between bactrian camel and animals in Vertebrata (chicken and zebrafish; NCBI genome accession codes GCF_000002315.3 and GCF_000002035.4), Mammalia (human, chimpanzee, mouse and rat; NCBI genome accession codes GCF_000001405.21, GCF_000001515.5, GCF_000001635.20 and GCF_000001895.4), Laurasiatheria (dog and horse; NCBI genome accession codes GCF_000002285.3 and GCF_000002305.2) and Artiodactyla (cattle and pig; NCBI genome accession codes GCF_000003055.4 and GCF_000003025.5). ( b ) Length of syntenic regions on each scaffold (Mb, million base pairs). Coverage is calculated as the length of syntenic region divided by the length of scaffold. Scaffolds with coverage >75%, >50% and <50% are represented by red, green and grey dots, respectively. ( c ) Supertree inference for nine mammals. The topology was evaluated by input tree bootstrap percentages. Distances are shown in millions of years. ( d ) Points represent pairs of medians of dN/dS ratios in camels and in cattle by KEGG pathways. Pathways in which rapidly evolving genes are significantly enriched (FDR<0.05) in camels and cattle are coloured in red and green, respectively. MAPK, mitogen-activated protein kinase; mTOR, mammalian target of rapamycin; TCA, tricarboxylic acid cycle. Full size image We constructed a phylogenetic tree with the supertree method [24] , using 2,345 single-copy orthologs among the animals ( Fig. 1c ). As shown in this tree, cattle and pig are the closest relatives of bacterian camels. All of them belong to Artiodactyla (even-toed ungulates) in taxonomy, which form a sister group with the clades of Perissodactyla (for example, horse) and Carnivora (for example, dog). This phylogeny was also consistent with previous evolutionary studies based on a smaller number of camel genes [25] . Among the single-copy orthologs, we further selected 332 orthologs with constant evolutionary rates to determine the time of speciation events. We estimated that cattle and bactrian camel lineages diverged about 55–60 million years ago (Mya) ( Fig. 1c and Supplementary Fig. S6 ), in the later Palaeocene period (55.8–65.5 Mya). This is slightly earlier than the first fossil evidence of the Camelidae family in North America (50 Mya) [26] . Rapidly evolving genes Rapid divergence of protein-coding genes, as measured by an increased ratio of nonsynonymous-to-synonymous substitutions (dN/dS), may have important roles in species differentiation and adaption [27] , [28] . We estimated the dN/dS ratios by the PAML package [29] for the camel and its closest cattle orthologs, taking the human ortholog as an outgroup. We used the likelihood ratio test (LRT) to identify 2,730 significantly faster evolving genes in camels than in cattle (false discovery rate (FDR)<0.05) and mapped them to the KEGG pathways ( Supplementary Table S7 ). It was shown that those rapidly evolving genes are significantly enriched in carbohydrate metabolism, lipid metabolism and signalling pathways regulating the metabolic processes, such as insulin (FDR=9.1 × 10 −4 ) and adipocytokine signalling pathways (FDR=0.03, Fig. 1d ). The accelerated evolution of these pathways involved in metabolism may help camels to optimize their energy storage and production in the desert. Characterization of heterozygosity We identified 1,986,420 heterozygous single nucleotide polymorphisms (SNPs) in the wild camel genome and 2,129,442 heterozygous SNPs in the domestic camel genome ( Supplementary Table S8 ). In both cases, the heterozygosity rates are estimated to be about 1.0 × 10 −3 across the whole genomes ( Fig. 2a ). The number of small indels identified in the two genomes is also comparable ( Supplementary Table S9 ). 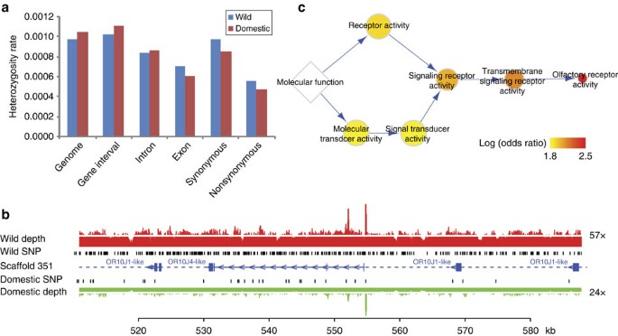Figure 2: Comparison of genetic diversity between wild and domestic bactrian camels. (a) Heterozygosity rate in coding and non-coding regions. The heterozygosity rate is calculated as the number of heterozygous SNPs divided by the length of corresponding genomic regions. (b) A genomic region where the heterozygosity of the domestic camel is significantly lower than that of the wild one. The region also contains a cluster of olfactory receptors (OR10J1, olfactory receptor 10J1). Genes and gene intervals are represented by solid and dash lines, respectively. Exons are shown in blue blocks and transcriptional directions are indicated by arrows. The locations of SNPs are marked in black. Sequencing depth in the region is also shown, with white lines indicating the average sequencing depth. (c) Enrichment of molecular function for genes with low heterozygosity in the domestic camel. The hierarchy of the Gene Ontology is displayed. The size of the circle is proportional to the number of genes in the genome, and the colour indicates the odds ratio of the enrichment. Figure 2: Comparison of genetic diversity between wild and domestic bactrian camels. ( a ) Heterozygosity rate in coding and non-coding regions. The heterozygosity rate is calculated as the number of heterozygous SNPs divided by the length of corresponding genomic regions. ( b ) A genomic region where the heterozygosity of the domestic camel is significantly lower than that of the wild one. The region also contains a cluster of olfactory receptors ( OR10J1 , olfactory receptor 10J1). Genes and gene intervals are represented by solid and dash lines, respectively. Exons are shown in blue blocks and transcriptional directions are indicated by arrows. The locations of SNPs are marked in black. Sequencing depth in the region is also shown, with white lines indicating the average sequencing depth. ( c ) Enrichment of molecular function for genes with low heterozygosity in the domestic camel. The hierarchy of the Gene Ontology is displayed. The size of the circle is proportional to the number of genes in the genome, and the colour indicates the odds ratio of the enrichment. Full size image We then classified the SNPs according to the gene annotations and calculated the heterozygosity rates for coding and non-coding regions ( Fig. 2a and Supplementary Table S10 ). Comparing with the wild camel, we found that an overall lower heterozygosity rate exists in the exon regions but not in other parts of the domestic camel genome, suggesting an artificial selection for certain genes in the domestic species [30] . As strong artificial selection would reduce genetic diversity around a locus (selective sweep) [31] , it was worth inspecting the genes and their functions in such a locus. We therefore used 10-kb windows to scan the genome to identify regions where the heterozygosity rate of the domestic camel is significantly lower than the wild one ( P <0.05 after Bonferroni correction, χ 2 -test) ( Fig. 2b ). There are 2,816 such regions identified, which incorporate 196 complete genes ( Supplementary Table S11 ). GO analysis of these genes showed that they are significantly enriched in membrane receptors and signalling transduction, and more specifically, olfactory receptor activity (FDR=3.8 × 10 −15 ) ( Fig. 2c and Supplementary Table S12 ). All of the olfactory receptors identified here (37 genes in total) are distributed in 17 different large scaffolds with median length over 800 kb ( Supplementary Table S11 ), implying that the loci for the olfactory receptors are independent in genealogy. Therefore, it is reasonable to compare the heterozygosity rates of these loci between the wild and domestic camels, even though we only obtained data from one individual of each type. These results suggested that olfaction may be an important object of artificial selection during the domestication of bactrian camels. Blood glucose levels In general, blood glucose levels in domestic ruminants (2.5–3.5 mmol l −1 ) are lower than in monogastric animals (3.5–5.0 mmol l −1 ) [32] , [33] . Although camels belong to the suborder Tylopoda within Artiodactyla , they are also ruminating herbivores with an extensive forestomach. The levels of blood glucose in camels (6–8 mmol l −1 ), however, are much higher than in most monogastrics [32] , [33] . Previous physiological experiments demonstrated that the high level of blood glucose in camels may be caused by their strong capacity for insulin resistance [33] . Consistent with this argument, our analysis shows that a large number of rapidly evolving genes in camels are involved in Type II diabetes mellitus (KEGG pathway accession code 04930) and the insulin signalling pathway (KEGG pathway accession code 04910) ( Fig. 1d ). The binding of insulin (INS) to insulin receptors could lead to tyrosine phosphorylation of insulin receptor substrates (IRSs), which will in turn activate PI3K and AKT to trigger downstream actions to promote glucose uptake and storage [34] , [35] ( Fig. 3a ). Of particular note was that PI3K and AKT , two critical genes in the process, have undergone rapid divergence in camels, which may change their responsiveness to insulin. Several other rapidly evolving genes, such as JNK , IKK , mTOR and ERK , could also result in insulin resistance via serine phosphorylation of IRS proteins to negatively regulate IRS activities [34] , [35] ( Fig. 3a ). 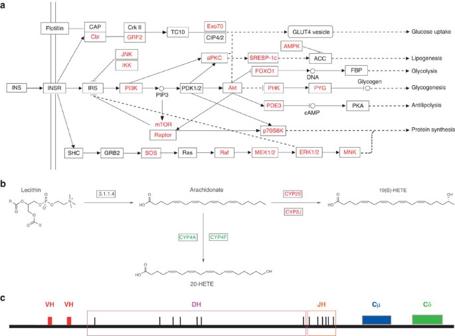Figure 3: Biological findings from the genome analysis. (a) The type II diabetes mellitus and insulin signalling pathway. The rapidly evolving genes in camels (shown in red) are identified in the pathway. Abbreviations, annotations and connexions are presented in accordance with KEGG standards: solid lines represent direct relationships among proteins (boxes) and metabolites (circular nodes), dashed lines represent indirect relationships, lines with arrowheads denote activation, and lines with the crossing mean inhibition. (b) The pathway of arachidonate synthesis and conversion. Arachidonate is synthesized from lecithin by PLA2G (EC: 3.1.1.4), and converted into 19(S)-hydroxyeicosatetraenoic acid (19(S)-HETE) by CYP2E and CYP2J (expansion in camel), or transformed into 20-hydroxyeicosatetraenoic acid (20-HETE) by CYP4A and CYP4F (contraction in camel). (c) The schematic diagram of IgH loci in the camel genome inferred from a complete V-D-J-C gene cluster in scaffold 355.1. Figure 3: Biological findings from the genome analysis. ( a ) The type II diabetes mellitus and insulin signalling pathway. The rapidly evolving genes in camels (shown in red) are identified in the pathway. Abbreviations, annotations and connexions are presented in accordance with KEGG standards: solid lines represent direct relationships among proteins (boxes) and metabolites (circular nodes), dashed lines represent indirect relationships, lines with arrowheads denote activation, and lines with the crossing mean inhibition. ( b ) The pathway of arachidonate synthesis and conversion. Arachidonate is synthesized from lecithin by PLA2G (EC: 3.1.1.4), and converted into 19(S)-hydroxyeicosatetraenoic acid (19(S)-HETE) by CYP2E and CYP2J (expansion in camel), or transformed into 20-hydroxyeicosatetraenoic acid (20-HETE) by CYP4A and CYP4F (contraction in camel). ( c ) The schematic diagram of IgH loci in the camel genome inferred from a complete V-D-J-C gene cluster in scaffold 355.1. Full size image Cytochrome P450 families Genes in cytochrome P450 (CYP) families are involved in the metabolism of arachidonic acids (KEGG pathway accession code 00590). For the CYP genes that were identified by InterProScan in the camel genome, we further assigned them to subfamilies by searching against the KEGG protein database and NCBI NR database. We found that the distribution of CYP genes in several subfamilies is quite different between the camel and other mammals ( Supplementary Table S13 ). In bactrian camels, there are 11 copies of CYP2J and 2 copies of CYP2E , more than in cattle (four and one, respectively), horses (one and one) and humans (one and one). In contrast, there are only one copy of CYP4A and two copies of CYP4F in camels, fewer than in cattle (three and seven, respectively), horses (three and seven) and humans (two and six). CYP2E and CYP2J can help to transform arachidonic acid into 19(S)-HETE, whereas CYP4F and CYP4A help to transform it into 20-HETE ( Fig. 3b ). 19(S)-HETE has been demonstrated to be a potent vasodilator of renal preglomerular vessels that stimulate water reabsorption [36] . So more copies of CYP2E and CYP2J and fewer copies of CYP4A and CYP4F may help camels produce more 19(S)-HETE, potentially useful for survival in the desert. In addition, the activity of CYP2J2 is regulated by high-salt diet and its suppression can lead to high blood pressure [37] . Camels are known to be able to take in a large amount of salt apparently without developing hypertension, perhaps because they have more copies of CYP2J genes. Heavy-chain antibodies A HCAb is an immunoglobulin that consists of only two heavy chains (IgH) and lacks the two light chains usually found in conventional Abs [8] . Camelids, such as camels, dromedaries and alpacas, are the only mammals that produce HCAbs. We searched the bactrian camel genome using the sequences of human, alpaca and dromedary IgH genes. In total, 17 VH (heavy-chain variable region), 7 DH (diversity region), 6 JH (joining region) and 10 CH (constant region) genes were identified in 16 scaffolds ( Supplementary Table S14 ). On the basis of a unique gene cluster in scaffold 355.1, we inferred an organization of the IgH loci similar to the typical mammalian Vn-Dn-Jn-Cn translocon [38] ( Fig. 3c ). It has been reported that amino-acid substitutions in the sites of 37, 44, 45 and 47 in the FR2 region of VH genes can result in conformational changes of the heavy chains, making them no longer able to bind to the light chains [39] . We found that five of the VH genes in the bactrian camel contain such mutation sites, which may code for HCAbs ( Supplementary Table S15 and Supplementary Fig. S7a ). A total of six Cγ genes were identified in bactrian camels, two of which have a ‘GT’ to ‘AT’ mutation on the donor splicing site in the CH1 region ( Supplementary Table S15 and Supplementary Fig. S7b ). This leads to another hallmark of the HCAbs—the lack of CH1 regions [40] . Our comparative analysis based on the genome sequences provides important insights into the evolution and domestication of bactrian camels. In addition, the identified genes and pathways may enhance our understanding of the genetic mechanisms that enable camels to survive in extreme environments. Further studies could focus on the molecular functions of the potential genes necessary for the special physiology of camels. These findings may also improve our understanding of metabolism-related diseases, thereby benefiting human health. Sampling, genome sequencing and assembly An 8-year-old male wild bactrian camel named ‘Naran’ was selected for the wild camel sequencing on 18 February 2010. The pedigree shows that it is from a pure bred wild camel group living in the Mongolian Wild Camel Protection Area, Bayan Tooree, Altai province, Mongolia. A 6-year-old male Alashan domestic bactrian camel from Altan ovoo balgas, Alshaa aimag, Inner Mongolia, China, was selected for the domestic camel sequencing on 8 March 2010. The blood from the ear tissue was collected for both bactrian camels. The genomic DNA was extracted using Puregene Tissue Core Kit A (Qiagen). The 500-bp paired-end and 3-kb mate-pair DNA library were sequenced on the Illumina Genome Analyzer IIx system. The 10-kb mate-pair DNA library was sequenced on the Applied Biosystems SOLiD 3 system. The 20-kb mate-pair DNA library was sequenced using the Roche Genome Sequencer FLX system. Library preparation, sequencing and base calling were performed according to the manufacturer’s recommendations. The genome sequence of the wild camel was assembled using SOAPdenovo [9] ( http://soap.genomics.org.cn ). We first assembled the reads with the insert size of 500 bp into contigs using the sequence overlap information, and then used the mate-pair libraries, step by step from the shortest to the longest insert size, to join the contigs into scaffolds. To fill the intra-scaffold gaps, we retrieved read pairs that had one read well-aligned on the contigs and the other read located in the gap region. We estimated the genome size of the wild bactrian camel based on the frequency distribution of the 17 base oligonucleotides. The reads with the insert size of 500 bp were used in this analysis. The occurrences of 17-mer in the reads were counted by Jellyfish [41] . The peak of the k-mer frequency ( M ) in reads is correlated with the real sequencing depth ( N ), read length ( L ) and k-mer length ( K ) according to the formula [42] M = N × ( L − K +1)/ L . We divided the total length of all reads by the real sequencing depth, and obtained an estimated genome size of 2.38 Gb. We also collected the C values and genome sizes of other mammals to estimate the genome size of camel ( http://www.genomesize.com ). The camel genome has a C value between 2.41 and 2.86 picograms, which is translated to a genome size between 2.02 and 2.40 Gb. Genome annotation The repeat sequences were identified by RepeatMasker (version 3.2.9) ( http://www.repeatmasker.org ) against the Repbase4 TE library (version 2009-06-04). The transfer RNAs (tRNAs) were predicted by tRNAscan-SE-1.23 (ref. 43 ), and short interspersed element-masked tRNAs and pseudo-tRNAs were eliminated. The ribosomal RNAs (rRNAs) were identified by aligning the eukaryote rRNA sequences from the SILVA [44] database using BlastN [45] with the cutoff of e value <1 × 10 −5 , identity >85% and match length >50 bp. The microRNAs (miRNAs) were identified by aligning the miRNA precursor sequences from miRBase [46] using BlastN with the cutoff of e value <1 × 10 −3 , identity >90% and match length >70 bp. As a result, 1701 tRNAs, 602 rRNAs and 330 miRNAs were identified in the camel genome. For protein-coding gene annotation, ab initio prediction was performed by Augustus [16] and GenScan [17] . Augustus predicts 26,842 genes, averaging 7.0 exons per gene. The average gene length is 21,269 bp, including coding regions 1,144 bp. GenScan predicts 42,677 genes, averaging 7.8 exons per gene. The average gene length is 31,880 bp, including coding regions 1,212 bp. Homology-based prediction was performed by searching against other mammalian gene sequences by genBlastA [47] . A reference gene set was created by merging all of the gene sets using EVidenceModeler [48] . We utilized InterProScan (v 4.3) [22] to collect domain information and GO terms of the camel proteins. We utilized KAAS [49] (KEGG Automatic Annotation Server) for KEGG pathway annotation. Comparative genomics and evolutionary analysis We performed BlastP [45] for all the camel proteins against the NCBI HomoloGene database [23] to assign them to gene families. To avoid too short local alignments, the best hit should have the e value <1 × 10 −5 and coverage length longer than 1/3 on both aligned proteins. The syntenic maps between the camel and other mammalian genomes were constructed by CHSMiner [50] , with their orthologs as anchor points. The gap size between two neighbouring ortholog pairs was set to be <2.0 Mb. Only the syntenic blocks with P -value less than 5 × 10 −5 were preserved. We used ClustalW [51] to perform multiple alignment for proteins in each ortholog family. The phylogeny tree was constructed based on the single-copy families in mammals, with chicken proteins as outgroups. The maximum likelihood tree for each family was built by Phylip [52] under the JTT model. The consense programme in Phylip was used to integrate the individual gene trees to the final supertree. To evaluate the supertree topology, we applied the bootstrap strategy to resample from the original tree set for 100 times [53] . On the basis of reconstructed mammalian supertree, we estimated the evolutionary time scales by PAML [29] . We used the rooted tree with the molecular clock assumption as the null hypothesis, and the unrooted tree without the assumption as the alternative hypothesis. The LRT was used to filter genes with substitution rate significantly deviated from the molecular clock assumption ( P <0.05). The remaining gene trees were calibrated with the divergence time points that are consistent between fossil and molecular evidence, i.e., human-chimpanzee: 5.5 Mya, human-cattle 94 Mya and mammal-bird: 310 Mya [54] . The codon-level alignment of CDS sequences from human, cattle and camel was performed by RevTrans [55] . Afterward, the codeml programme in PAML [29] was applied to estimate the dN/dS ratio for each gene. To select the rapidly evolving genes in camels, we used the model that the branches of camel and cattle have the same dN/dS ratio as the null hypothesis, and the model that all branches have free dN/dS ratios as the alternative hypothesis. The LRT was used to select rapidly evolving genes in the camel lineage (FDR<0.05). SNP and heterozygosity analysis We utilized the BWA program [56] to remap the usable reads from the wild and domestic camel to the assembled scaffolds, respectively. The parameters for mapping were chosen as the seed length of 28 and the maximum occurrences for extending a long deletion of 20. The reads that could map to multiple positions were removed in the following analysis. The candidate SNPs and small indels (<50 bp) were retrieved by the SAMtools pipeline [57] with default settings. We flagged a candidate SNP as a likely false-positive one if it exhibits the following behaviour: (1) total depth is above 400 or below 10; (2) root mean square of mapping quality is below 20; (3) depth of alternate bases is below 4; (4) P -value of reference and non-reference bases being evenly distributed on both strands is below 1 × 10 −4 (Fisher exact test). These thresholds were applied to both the heterozygous SNPs within the wild and domestic camel genome, and the homozygous SNPs between them. The heterozygosity rate was estimated as the density of heterozygous SNPs for the whole genome, gene intervals, introns and exons, respectively. For the estimation of local heterozygosity rate, sliding windows of 10 kb that had 90% overlap between adjacent windows were used to scan the genome. The χ 2 -test was performed for each window to identify the regions where the heterozygosity rate of the domestic camel is significantly lower than that of the wild one ( P <0.05 after Bonferroni correction). The GO enrichment analysis for genes located in the regions was performed by GOEAST [58] . Accession codes : This Whole Genome Shotgun project has been deposited in DDBJ/EMBL/GenBank as project accession PRJNA76177 . The genome assembly has been deposited in DDBJ/EMBL/GenBank under the accession code AGVR00000000 . The version described in this paper is the first version, AGVR01000000. How to cite this article : Jirimutu. et al . Genome sequences of wild and domestic bactrian camels. Nat. Commun . 3:1202 doi: 10.1038/ncomms2192 (2012).